Computational design of self-assembling register-specific collagen heterotrimers The contribution of pairwise amino-acid interactions to the stability of collagen triple helices has remained elusive. Progress in this area is critical for the prediction of triple helical stability from sequences and the preparation of mimetic materials based on this fold. Here we report a sequence-based scoring function for triple helices that takes into account the stability conferred to collagen by axial lysine–aspartate salt bridges. This function is used to predict the stability of a specific register formed from three distinct peptide sequences and that of all alternative compositions and registers. In the context of a genetic algorithm we use it to select sequences likely to self-assemble with high stability and to the exclusion of the other 26 possible combinations. We validate our methodology by synthesis and structural characterization of the designed peptides, which self-assemble into a highly stable ABC triple helix with control over both composition and register. Proteins have mastered the cooperative use of non-covalent interactions to self-assemble into complex three-dimensional architectures. A stringent test of our understanding of the principles that determine a protein's structure from the physicochemical information encoded in its amino-acid sequence lies in the design of synthetic polypeptide chains that are able to replicate this feat; that is, to accurately fold into a particular conformation while avoiding the population of closely related states. Computational design protocols have been successful at this task, particularly when dealing with globular proteins [1] , [2] , [3] and α-helical coiled coils [4] , [5] , [6] . These structural motifs benefit from the presence of a hydrophobic core that is buried on exposure to an aqueous environment and acts as a major driving force in the folding and association of the peptide chains [7] . A structural motif that, despite its predominance in higher organisms, has seen rather limited success in this field is the collagen triple helix [8] , [9] . The large number of competing states that need to be explicitly modelled and the fact that only solvent-exposed amino acids can be used to bias the chain association in this fold, make it a challenging system for de novo design. Collagenous domains are characterized by long uninterrupted stretches of three amino-acid repeats of the form X-Y-G. Proline is the most abundant residue in the X position of proteins in this family and 4R-hydroxyproline (single letter code O), a posttranslationally modified amino acid with a hydroxyl group in the γ-carbon of the proline side chain, is the most abundant residue in the Y position. P and O have a preference for distinct conformations of the pyrrolidine side chain that biases the main chain φ dihedrals to values close to those found in the X and Y positions of the triple helix, thus reducing the unfavourable conformational entropy change on the assembly of the unfolded chains [10] . The glycine residues, present at every third position in the sequence, pack tightly in the core of the helix forcing the peptide chains to self-assemble with a one amino-acid stagger between adjacent strands. This arrangement enables the canonical hydrogen-bonding network of this super-secondary structure, which goes from the amide proton of glycine in one strand to the carbonyl of the amino acid in the X position of the following strand [11] . It is possible to synthesize short peptide sequences that self-assemble into highly stable homotrimeric triple helices following these sequence requirements. Such peptides, usually referred to as collagen mimetic peptides (CMPs), have been widely used to study the relationship between amino-acid composition and triple helical stability [12] , [13] , [14] , folding rate [15] , [16] , [17] and super-helical symmetry [18] , [19] , [20] , as well as to identify ligand-binding motifs [21] , [22] , [23] and provide the structural basis for their recognition [24] , [25] , [26] . Self-assembling heterotrimeric CMPs are not straightforward to synthesize with high specificity. Because of the one residue stagger induced by the packing requirements, different helical registers are possible for a given heterotrimeric composition depending on the chemical identity of the leading, middle and lagging chains. Furthermore, when dealing with mixtures of peptides, several helical compositions are also possible. For example, a mixture of two sequences (A and B) can form a total of eight distinct triple helices: two homotrimers (A 3 and B 3 ) and two distinct heterotrimers (A 2 B and AB 2 ) with three unique registers for each heterotrimeric composition. A ternary mixture can populate a total of 27 distinct helices, including 6 distinct registers of the ABC heterotrimer ( Fig. 1 ). This problem has hampered the success of both rational [27] , [28] , [29] , [30] and computational design [8] , [9] strategies to generate self-assembling heterotrimeric triple helices with control over both the helical composition and chain stagger. The most successful computational approach thus far was developed by Nanda and group [9] and used a sequence-based scoring function adapted from coiled-coil design and a simulated annealing Monte Carlo search algorithm. Their methodology focuses on the problem of compositional control in ABC-type heterotrimers, and the resulting triple helices are less stable than those with comparable specificity achieved through rational design [30] . A system with control over both composition and register is highly desirable as it can be used to extend the work done with homotrimeric CMPs to the heterotrimeric collagens [31] . 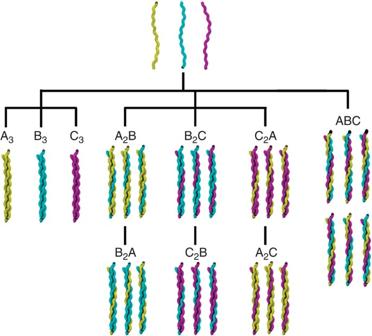Figure 1: Schematic representation of the triple helices that can potentially form. In total, ten compositions form. Each composition with two distinct peptides can form three registers while the ABC composition can form six for a total of 27 unique combinations. Figure 1: Schematic representation of the triple helices that can potentially form. In total, ten compositions form. Each composition with two distinct peptides can form three registers while the ABC composition can form six for a total of 27 unique combinations. Full size image At first glance it may appear that the difference between registers in a particular triple helical composition is of minor significance, as it seems that only the order of the peptide chains is altered. However, the three-dimensional presentation of chemical functionality (the amino-acid side chains) is entirely changed and is unique for each register. This is of critical importance for the understanding of collagen's interaction with itself (fibrillogenesis) as well as its recognition by other extracellular matrix proteins in processes as varied as degradation, cell migration, differentiation and metastatis. Here we describe a multistate computational design protocol using a sequence-based scoring function that exploits recently derived sequence–structure relationships [14] between oppositely charged amino acids within the triple-helical fold. This approach allows us to explicitly calculate all the possible triple helical states within a peptide mixture and optimize the stability of the desired target state while maximizing the energy gap between the target and the most stable decoy. As a proof of principle, we use this methodology to design three peptides that fold into an ABC heterotrimer. Using circular dichroism (CD) polarimetry and nuclear magnetic resonance (NMR) spectroscopy, we show that the resulting triple helix is both stable and specific towards the target state. Computational design There are two main components to any computational protein design protocol: an energy function that is able to accurately assess the stability of a given structure and a search algorithm that efficiently searches the sequence space of interest. In the subsequent sections we will describe our approach to both components in the context of heterotrimeric triple helical design. Although our methodology is general and can be used to generate any type of collagen heterotrimer, we tackle the most complex problem with the largest number of competing states, the self-assembly of a register-specific ABC heterotrimer. Following the sequence selection algorithm, we show that the designed peptide chains indeed self-assemble into the desired ABC heterotrimer with the correct chain registration using NMR and high thermal stability, as evidenced by CD melting studies, while avoiding the formation of any of the remaining 26 competing states. We developed a sequence-based scoring function for triple helical proteins based on our understanding of the non-covalent interactions that stabilize this protein fold. We set the prototypical homotrimeric sequence, (POG) 10 , as the reference state and gave its stability a numerical value of 0 in our relative scale. Single point mutations with respect to this scaffold, which are known to be destabilizing [13] , are given a positive numerical value. Pairs of amino acids that are known to interact favourably and stabilize the fold [32] are given negative numerical value. In principle any single and double substitutions can be allowed, but we have restricted ourselves to oppositely charged amino acids, particularly, lysine and aspartic acid, as they have shown to engage in the most stabilizing interchain ionic hydrogen bonds in the context of rationally designed collagen heterotrimers [27] . Furthermore, we restrict the amino-acid identity of the X position to either P or D and that of the Y position to either O or K following the pattern observed in naturally occurring collagens, in which negatively charged amino acids have higher propensity for the X position and positively charged amino acids have a higher propensity for the Y position [12] . Even in this reduced space, two distinct contact geometries between the oppositely charged amino acids are possible, which we refer to as lateral and axial interactions [14] . Our previous analysis of structural, biophysical and computational data indicates that lateral contacts are only marginally stabilizing in triple helices [14] , [33] , while axial contacts have been shown to effectively bias self-assembling peptides towards a specific heterotrimeric target state [30] , thus only the axial geometry was considered in our current approach. With these considerations in mind, the energy score ( E ) of a particular sequence is given by where M is the number of ionizable residues, N is the number of axial salt bridges and and their respective contributions. 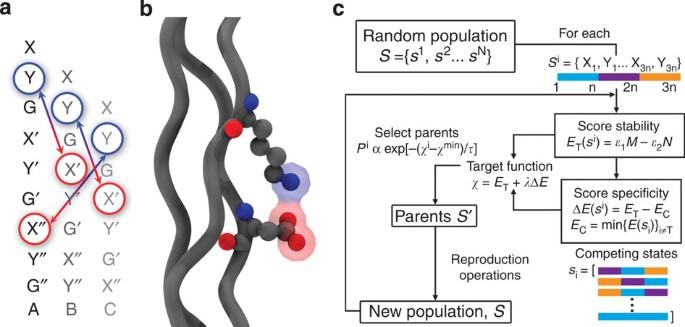Figure 2: Interchain interactions and computational design protocol. (a) Relative sequence position of the Lys-Asp axial interactions necessary to stabilize the triple helix. (b) Molecular representation of the contacts shown ina(from pdb id 3U29). (c) Schematic of our sequence selection genetic algorithm. Each coloured bar represents a string that encodes a peptide's amino-acid sequence, with cyan being the leading strand, purple the middle strand and orange the lagging strand in the target ABC heterotrimer. Figure 2a shows the relative position of interacting amino acids in axial salt bridges in terms of aligned triple helical sequences, and Fig. 2b is a molecular representation of the interacting side chains. We hypothesize that this function, despite its simplistic form and the numerous approximations used in its formulation, captures the dominant contributions to the free energy difference between triple helical states in the sequence space of interest by penalizing point mutations from the POG template and rewarding double mutations that lead to the formation of ionic hydrogen bonds between adjacent strands. We have observed that the energy penalty associated with the presence of aspartate and lysine residues in the X and Y positions of a collagen triple helix is approximately equal to the stability gain through the formation of an axial salt-bridge. Therefore we set to 1 and to 2. Furthermore, although we arrive at our expression using intuitive supramolecular considerations, it can be independently derived using a rigorous theoretical approach. It can be shown that equation (1) corresponds to a truncated, simplified version of the cluster expansion, recently applied by Keating and group [34] , to evaluate protein energies from their amino-acid sequences ( Supplementary Information ). Figure 2: Interchain interactions and computational design protocol. ( a ) Relative sequence position of the Lys-Asp axial interactions necessary to stabilize the triple helix. ( b ) Molecular representation of the contacts shown in a (from pdb id 3U29). ( c ) Schematic of our sequence selection genetic algorithm. Each coloured bar represents a string that encodes a peptide's amino-acid sequence, with cyan being the leading strand, purple the middle strand and orange the lagging strand in the target ABC heterotrimer. Full size image The second component of the design protocol is a search algorithm that is able to explore the space of interest and select sequences that satisfy a given set of constraints. We use a genetic algorithm (GA) for this purpose as it has been successful in multistate protein design problems [35] , [36] . For this approach, a fitness function needs to be defined and optimized. We define our fitness function, χ , as where E T represents the stability of the target state, λ is a proportionality constant and Δ E is the difference in stability between the target state and the most stable member of the competing state ensemble, which is a measure of the specificity of the system towards the target state. The first term biases the search towards sequences that have low energy scores and thus a large proportion of paired charged amino acids or a high content of proline and hydroxyproline residues. The second term biases the search towards sequences where there are more unpaired basic and acidic residues in the most stable competing state than in the target structure. In our GA ( Fig. 2c ) we start with a random population of sequences that are scored according to their fitness. A second subset is generated that is augmented with some of the fittest members of the initial population, which are then subjected to reproduction operations to generate an offspring generation. This process is repeated until a target fitness is met or a preset number of generations is produced. Details on the GA are available in the Methods section. The best fitness score found for ABC-type sequences was −12; this means that there are 12 more unpaired ionizable residues in the most stable competing state than in the desired triple helix. This solution is not unique (see Supplementary Table S1 for ten additional triple helices with the same fitness) and although we cannot prove that it corresponds to the global minimum of the fitness function, we show experimentally that it is sufficient to preclude the self-assembly of any alternative states when all three sequences are present in solution. Experimental characterization Table 1 shows the three sequences that were selected for experimental characterization, which will be referred to as α, β and γ respectively. These peptides have smaller net charge (−2, +2 and 0, respectively) than the rationally designed triple helical heterotrimers previously studied in our laboratory despite having a higher proportion of charged residues. There are 14 possible axial contacts, which are satisfied in the desired register, α·β·γ, giving it a stability score of 0. The next most stable configuration corresponds to eight paired salt bridges with 12 unpaired ionizable residues and there are several triple helices with that arrangement: 2 alternative ABC registers (β·γ·α and γ·α·β) and 10 AAB-type helices (α·α·β, α·β·α, α·β·β, β·α·β, α·α·γ, α·γ·γ, β·γ·γ, γ·β·γ, β·γ·β and β·β·γ). Table 1 Peptide sequences and abbreviations. Full size table To assess the performance of our GA, samples were prepared for CD melting studies with a total peptide concentration of 0.3 mM in 10 mM phosphate buffer at pH 7. Peptides were slowly heated while monitoring elipticity at 225 nm. We utilize the minimum in the first derivative of the unfolding curve to define the melting temperature in our analysis. Each sequence was examined individually, in 1:1 binary mixtures and in a 1:1:1 ternary mixture (all experiments are available in Supplementary Fig. S1 ). Only peptide-γ shows the formation of a homotrimeric helix under the examined conditions, as evidenced by the weak cooperative transition observed in the unfolding experiment. All binary mixtures show cooperative transitions with the 1:1 α/β mixture having the lowest molar residual ellipticity (MRE) and melting temperature ( T m ). The 1:1 α/γ and β/γ mixtures both show transitions with the same T m (43 °C, Fig. 3 ) and comparable MRE. The ternary mixture shows the highest T m of the system with an unfolding transition at 58 °C, 15 °C higher than the most stable competing AAB heterotrimers ( Fig. 3 ). We attribute this difference in thermal stability to the difference in the number of charge pairs between the desired register and the AAB competing states. Although this result is encouraging, the presence of competing states can be easily masked in CD melting studies. Furthermore, this technique cannot differentiate between different registers of a given helix to show that the cooperative transition observed in the ternary mixture indeed corresponds to the designed register. For this reason solution NMR studies were carried out to corroborate that the ternary mixture, within the detection limits of NMR, is indeed composed solely of the desired α·β·γ heterotrimer. 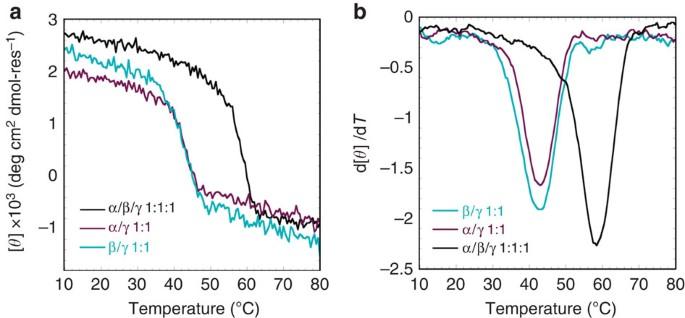Figure 3: Circular dichroism melting studies. (a) Melting profiles for the ternary mixture (target state—black) and the two most stable binary mixtures (competing states—red and cyan). (b) First derivate of the melting curve with respect to temperature for the ternary mixture (target state—black) and the two most stable binary mixtures (competing states—red and cyan). Figure 3: Circular dichroism melting studies. ( a ) Melting profiles for the ternary mixture (target state—black) and the two most stable binary mixtures (competing states—red and cyan). ( b ) First derivate of the melting curve with respect to temperature for the ternary mixture (target state—black) and the two most stable binary mixtures (competing states—red and cyan). Full size image Samples for NMR were prepared in 10 mM phosphate buffer at pH 7 with 10% D 2 O. Once again, each sequence was examined individually, in 1:1 binary mixtures and in a 1:1:1 ternary mixture. 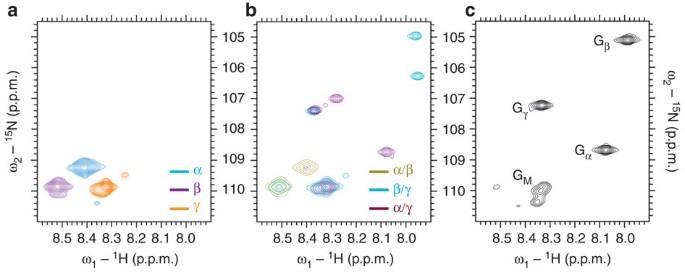Figure 4:1H,15N-HSQC spectra. (a) Overlaid spectra of the three samples containing individual peptides α, β and γ. (b) Overlaid spectra of the three samples containing binary mixtures α/β, β/γ and α/γ. (c) Spectrum of the annealed ternary mixture of α/β/γ. GMcorresponds to residual monomeric peptides, while Gα, Gβ, and Gγcorrespond to the labelled glycines of the triple helical species. Figure 4 shows the 1 H, 15 N-heteronuclear single quantum coherence (HSQC) spectra of the different samples at 37 °C. Each of the peptide sequences contains an 15 N-labelled glycine at position 15 to facilitate the analysis. A single peak is expected from every unique chemical environment that each of the peptides encounter. No homotrimeric triple helices are present at this temperature, as expected from the CD melting studies and evidenced by the absence of trimeric peaks originating from the samples containing a single sequence. The overlaid spectra of individual peptides, Fig. 4a , shows only the presence of broad monomeric peaks. Figure 4b showcases the overlaid spectra of the binary mixtures. The blue peaks correspond to the α/β mixture, which are identical to the peaks observed for the individual peptides, indicating the absence of α 2 β or αβ 2 trimers at this temperature. On the other hand, both the α/γ and β/γ mixtures show distinct trimeric peaks, green and red, respectively; these peaks correspond to the molecular fingerprint of the competing states of alternative composition and can be used to investigate their presence or absence from the ternary mixture. The annealed α/β/γ mixture shows only three distinct heterotrimeric cross-peak of equal intensity, as well as residual monomeric peaks. The three peaks in this spectrum ( Fig. 4c ) can be unambiguously assigned to the α, β and γ chains (Methods). These experiments corroborate the CD data and indicate that we indeed produce a single composition system, where competing states of alternative stoichiometry are not populated when all three peptide sequences are present. Figure 4: 1 H, 15 N-HSQC spectra. ( a ) Overlaid spectra of the three samples containing individual peptides α, β and γ. ( b ) Overlaid spectra of the three samples containing binary mixtures α/β, β/γ and α/γ. ( c ) Spectrum of the annealed ternary mixture of α/β/γ. G M corresponds to residual monomeric peptides, while G α , G β , and G γ correspond to the labelled glycines of the triple helical species. Full size image The last step required to validate our design protocol is to experimentally characterize the chain stagger or register of the three-peptide strands. For this purpose we use a 1 H, 1 H-nuclear Overhauser effect spectroscopy (NOESY)- 15 N-HSQC spectrum ( Fig. 5a ). To assign the relative stagger of the chains within the triple helix, observed interchain nuclear Overhauser effects (NOEs) need to be compared with expected NOEs from the different registers. In general, any two protons that are within ~5 Å can give rise to a cross-peak in the NOESY spectrum. We use this criterion and generated a list of expected NOEs for the following pairs of atoms in each of the six possible registers using a structural model and aligned sequences: G α 15(NH)–G β 15(NH), G β 15(NH)–G γ 15(NH), G γ 15(NH)–G α 15(NH), G β 15(NH)–O γ 14(Hα) and G β 15(NH)–K α 14(Hα). Table 2 shows a comparison of the observed NOEs in the H, 1 H-NOESY- 15 N-HSQC spectrum of the α/β/γ mixture and the expected cross-peak patterns for each of the registers. Discrepancies between the observed resonances and the expected ones are highlighted in red. Only one of the expected patterns, the one corresponding to the target state, matches the NOE data. It should be noted that to make the assignment, the lack of certain cross-peaks is taken as the absence of the supramolecular species that would give rise to the resonances. Although this can be a dangerous assumption, we utilize sets of peaks that are structurally equivalent in the different assemblies to mitigate concerns about the use of a negative result to make a conclusion. For instance the NH–NH cross-peaks that arise from the glycine packing at the core of the helix are observed between chains α and β as well as chains β and γ. The corresponding peak between chains α and γ is absent, but is structurally equivalent to the observed peaks in four of the six possible ABC registers (α·γ·β, β·γ·α, β·α·γ and γ·α·β). As we do not observe this resonance we rule out the presence of the four competing registers, in which chains α and γ are adjacent. To discriminate between the two remaining registers we use the G β 15(NH)–O γ 14(Hα), which is expected from the target state, α·β·γ, but not in the last alternative register: γ·β·α. We take this as evidence that the target state is present but it would also be consistent with the pattern arising from both species being present in solution. To rule out this possibility we look at the structurally equivalent correlation in the γ·β·α register: G β 15–K α 14. This peak is absent from the spectrum, which we take as an indication that the γ·β·α register is not present in the peptide mixture. 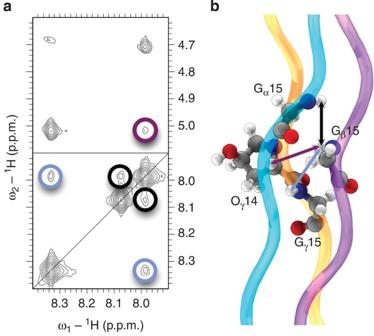Figure 5: Register determination. (a) 2D1H,1H-NOESY-15N-HSQC spectrum of the annealed ternary mixture at 37 °C highlighting amide-amide NOEs. (b)In silicomodel showing the backbone NOEs highlighted inawith the peptide-α coloured cyan, β in purple and γ in orange. Coloured circles inacorrespond to the coloured arrows inb. Figure 5: Register determination. ( a ) 2D 1 H, 1 H-NOESY- 15 N-HSQC spectrum of the annealed ternary mixture at 37 °C highlighting amide-amide NOEs. ( b ) In silico model showing the backbone NOEs highlighted in a with the peptide-α coloured cyan, β in purple and γ in orange. Coloured circles in a correspond to the coloured arrows in b . Full size image Table 2 Observed and expected NOEs for each of the six possible registers of the designed ABC heterotrimer. Full size table An in silico model in Fig. 5b shows the spatial arrangement of the amino acids utilized for register determination. Although the chemical shift of most charged amino acids cannot be unambiguously determined ( Supplementary Fig. S2 ), a combination of 1 H, 1 H-NOESY and two-dimensional (2D) 1 H, 1 H-NOESY- 15 N-HSQC spectra at 37 °C can be used to assign one of the axial salt bridges that stabilize our designed triple helix. Supplementary Fig. S3 shows the resonances used in the characterization of this interstrand interaction between K α 14 and D β 16. The chemical shift D β 16(NH) can be identified using the sequential NOE to the labelled G β 15(Hα) in the NOESY spectrum. There is also a clear resonance between D β 16(NH) and a lysine -methylene. Most -protons have comparable chemical shifts and thus the assignment can only be made considering the sequence, but this resonance is characteristic of K–D axial salt bridges and validates our design hypothesis by showing that axial salt bridges are indeed present in our system. This study presents a minimalistic approach to the design of heterotrimeric collagen-like peptides. By constraining the sequence space and understanding what amino-acid configurations are stabilizing and destabilizing for triple helices within those constraints, we are able to generate sequences that form ABC-type triple helices with a high-thermal stability and control over both the composition and the relative stagger of the peptide chains within the helix. Our automated sequence selection algorithm is successful because of the balance struck in our scoring function between the destabilization induced on triple helical assemblies by changing conformationally restricted imino acids to ionizable residues and the stabilization conferred on the formation of axial interstrand ionic hydrogen bonds. The scoring function we use is exceptionally simple and in principle, similar peptides could be designed by hand. However, the difficulty with designing by hand is that ever time a modification is made to the target state, all 26 competing states also need to be evaluated and the gap between the target and competing states assessed. A computational approach greatly simplifies this process and allows potential sequences to be generated in a few minutes on a personal computer. Our experimental characterization of the peptide sequences generated by the GA agree with the initial hypothesis that our minimalistic energy function captures the dominant contributions to the chemical potential of triple helical peptide mixtures within the set sequence constraints. Although other factors besides the formation of axial salt bridges, such as electrostatic repulsion and contributions of different single and double substitutions, could be incorporated to improve the accuracy of the model, their relative strength needs to be carefully weighted for triple helical systems. Nanda and group [9] recently used a comparable sequence-based scoring function adapted from coiled-coil design and a simulated annealing Monte Carlo search algorithm to tackle the problem of compositional control in ABC-type heterotrimers. Their study generated sequences with significantly lower thermal stability, ~30 °C, and does not differentiate based on register. Additionally, that study explored a larger sequence space by allowing lysine residues in the X position as well as aspartic acid residues in the Y position, relied on repulsion between amino acids of identical charge and weighted equally axial and lateral geometries between oppositely charged residues. We believe that the main reason for the difference in melting temperature between the two designed peptide systems lies in the fact that axial salt bridges dominate the energy landscape. If other interactions are to be included within the model, their relative contributions need to be weighted more effectively. Establishing proper weighting for additional pairwise interactions with collagen triple helices (both additional geometries and additional amino-acid types) is an important goal for full understanding of the structure and self-assemble of collagen helices, natural and synthetic. Currently, the registration process in heterotrimeric members of the collagen family, such as types I, IV and IX, is poorly understood. It is thought that globular domains capable of setting the composition have a dominant role in this process, but our synthetic analogue shows that it is indeed possible to control the composition and register of a triple helical system using information encoded solely in the collagenous domain. Our simple scoring function can be expanded to account for other amino acids, and their respective interactions, to study the stability and specificity profiles of natural heterotrimeric collagens and shed light on their registration mechanism and the role that triple helical domains have in that process. Finally, this methodology can be used to generate flanking regions for heterotrimeric host-guest peptide studies. The designed N- and C-terminal domains can be used to set the composition and chain register as well as drive triple helix formation, similar to POG triplets in homotrimers, and the guest domain can be used to include wild-type sequences or mutants opening a whole new chapter in the study of the biochemistry and biophysics of this important protein family. Scoring function Each triple helical sequence composed of 30 amino acids per chain is encoded as a 60-bit string, odd bits represents the X positions and even the Y positions, glycines are excluded as they are not designable amino acids in this context. Bits 1–20 represent chain A, 21–40 chain B and 41–60 chain C. Each sequence is scored according to equation (1) by counting the number of charged residues and axial salt bridges. The / ratio in (1) can be used to explore different regions in sequence space; however, we use a value of 1 for and 2 for , with the rationale that a paired salt bridge approximately cancels out the destabilization caused by the point mutations [32] . Genetic algorithm We start with a population of 80 random 60-bit strings. The fitness, χ , of each member of the population is calculated using the energy score of the sequence, the energy score of the most stable member of the competing state ensemble and a value of 1 for λ , the proportionality constant. This value was chosen with the rationale that both terms in the fitness function should be equally weighted as their absolute values have comparable magnitudes. The competing state ensemble is generated from the 26 remaining combinations of the three segments corresponding to chains A, B and C, as described in the scoring function section. A second population of identical size is generated by stochastically choosing members of the initial population with a probability, P , proportional to exp[-( χ − χ min )/ τ ], with τ =1. All members of this set are paired and a new generation is produced using variable, randomly selected, single crossover combinations of the parent sequences. During the crossover step if two identical sequences are chosen as parents, random single amino-acid mutations are performed with a probability P =0.5 to avoid early convergence on a local minimum. After this operation, stochastic single amino-acid mutations with a probability of 0.05 are performed to keep genetic variability. For the sequences reported here, the algorithm was run for 2,000 generations and the final sequence was stored. Peptide synthesis Peptides were synthesized with an Advanced Chemtech Apex 396 synthesizer using Fmoc solid-phase peptide chemistry and a Rink MBH amide resin. During the automated procedure, a manual addition of 15 N-labelled glycine, purchased from Cambridge Isotope Laboratories, was carried out in position 15. All peptides include a tyrosine (for concentration determination) and a glycine spacer at the C-terminus and are C-terminally amidated and N-terminally acetylated to eliminate any competing electrostatic interaction at the termini. The peptides were purified on a Varian PrepStar220 HPLC with a preparative reverse-phase C-18 column using a linear water/acetonitrile gradient each containing 0.05% trifluoroacetic acid and analysed by electro-spray ionization time of flight mass spectrometry on a Bruker microTOF instrument ( Supplementary Fig. S4 ). Sample preparation Concentration of stock solutions was determined by ultraviolet visible absorption at 275 nm using a molar extinction coefficient of 1,400 cm −1 M −1 . All peptide mixtures were prepared, annealed at 85 °C and incubated for a week at room temperature before experimental measurements were performed. Circular dichroism CD experiments were performed with a Jasco J-810 spectropolarimeter equipped with a Peltier temperature control system. Samples were prepared to a total concentration of 300 μM in 10 mM phosphate buffer at pH 7 by mixing the desired peptides in the appropriate ratio (1:1 for binary samples and 1:1:1 for the ternary sample). Spectra were acquired between 215 and 250 nm to locate the maximum near 222 nm, which was monitored during unfolding experiments. Melting curves were performed from 5 to 85 °C with a heating rate of 10° C h −1 . The first derivative of the melting curve was taken to determine the melting temperature ( T m ) of the sample, which we define as the minimum in the derivative graph. The MRE is calculated from the measured ellipticity using the equation: where θ is the ellipticity in mdeg, m is the molecular weight in g mol −1 , c is the concentration in mg ml −1 , l is the pathlength of the cuvette in cm, and n r is the number of amino acids in the peptide. Nuclear magnetic resonance NMR experiments were recorded in an 800 MHz Varian at 37 °C spectrometer equipped with a triple resonance probe. Samples were prepared at two different total peptide concentrations (1 mM for samples containing a single peptide and 3 mM for peptide mixtures) in a10 mM phosphate buffer at pH 7 and a 9:1 ratio of H 2 O to D 2 O. The spectra were processed using NMRpipe [37] and analysed using ccpnmr [38] . Each sample containing a mixture of peptides was characterized using 2D total correlated spectroscopy (TOCSY), NOESY, 1 H, 15 N-HSQC and 2D 1 H, 1 H-NOESY- 15 N-HSQC experiments while samples containing single sequences were characterized using 1 H, 15 N-HSQC spectra at 37 °C. Additional 1 H, 15 N-HSQC spectra for the ternary mixture were acquired at 5, 25 and 45 °C ( Supplementary Fig. S5 ). TOCSY spectra with a 50 ms spinlock duration at 8 kHz were acquired with a total of 1,700 complex points recorded in 8 scans for the directly acquired dimension, while 500 increments were used in the indirect dimension. NOESY spectra with a 100 ms mixing time were acquired with a total of 1,700 complex points recorded in 8 scans for the directly acquired dimension while 500 increments were used in the indirect dimension. A square spectral window of 1,000 Hz was used for all homonuclear spectra. For the 2D 1 H, 1 H-NOESY- 15 N-HSQC spectra, a mixing time of 100 ms was used and a total of 1,600 complex points in 32 scans for the direct dimension and 400 increments for the indirect dimension were acquired using a spectral window of 8,000 Hz for the direct dimension and 7,200 for the indirect dimension. A total of 1,208 complex points in 32 scans for the direct dimension and 100 increments in the indirect dimension were acquired for the 1 H, 15 N-HSQC experiments, using a spectral window of 10,000 Hz in the hydrogen dimension and 1,200 Hz in the nitrogen dimension. Square Cosine bell window functions were used as apodization functions, and the data were zero-filled to the next power of two in both dimensions. Drift and baseline corrections were applied when necessary. Sequential assignment The chemical shift of the labelled glycines (position 15 in each chain) was determined using a combination of 1 H, 15 N-HSQC, 1 H, 1 H-NOESY, 1 H, 1 H-TOCSY and 2D 1 H, 1 H-NOESY- 15 N-HSQC spectra at 37° C. Supplementary Figs S6–S8 show the resonances used in the assignment. In the case of peptide- α ( Supplementary Fig. S6 ), the chemical shift of K14(Hα) proton, K14(Hγ1) and K14(Hγ2) can be identified using the sequential NOE to the labelled G15(NH) in the 1 H, 1 H-NOESY- 15 N-HSQC spectrum as well as the intra-residue NOEs and TOCSY cross-peaks arising from the unlabelled lysine residue. Although the intra-residue peaks K14(Hγ1)–K14(Hγ2) and K14(Hγ1)–K14(Hα) in Supplementary Fig. S4a cannot be unambiguously assigned because most of the lysine side chains present similar shifts for the γ-methylene protons, their unique aliphatic chemical environment gives rise to a characteristic chemical shift that can be used to unequivocally identify the labelled glycine corresponding to the α-chain, as none of the remaining sequences have lysine residues preceding the labelled position. Similarly, in the case of peptide-β ( Supplementary Fig. S7 ), the chemical shift of O14(Hα) proton, O14(Hβ1), O14(Hβ2) can be identified using the sequential NOE to the labelled G15(NH) in the 1 H, 1 H-NOESY- 15 N-HSQC spectrum as well as the intra-residue NOEs and TOCSY cross-peaks arising from the unlabelled hydroxyproline residue, O14(Hβ1)–O14(Hα) and O14(Hβ2)–O14(Hα). The chemical shift of D16(NH) can be identified from the sequential D16(NH)–G15(Hα1) and D16(NH)–G15(Hα2) NOEs in the 1 H, 1 H-NOESY spectrum, these are necessary to differentiate sequences β(O 14 G 15 D 16 ) and γ(O 14 G 15 P 16 ). Finally, in the case of peptide-γ ( Supplementary Fig. S8 ) the chemical shift of O14(H α ) proton, O14(Hβ1), O14(Hβ2) can be identified using the sequential NOE to the labelled G15(NH) in the 1 H, 1 H-NOESY- 15 N-HSQC spectrum as well as the intra-residue NOEs and TOCSY cross-peaks arising from the unlabelled hydroxyproline residue, O14(Hβ1)–O14(Hα) and O14(Hβ2)–O14(Hα). Homology modelling A model of the α·β·γ register was prepared using the Rosetta software suite [39] using the crystal structure of a triple helical peptide (pdb id: 1K6F) as a template [40] . After mutating the residues using the fixed backbone design application, rounds of flexible backbone modelling using the backrub and side chain relaxation were carried out. Because this particular macromolecular software suite lacks explicit electrostatic scoring terms but includes directional hydrogen-bonding potentials, distance constraints were placed on the charged residues to bias them towards the axial salt bridge supported by the D(NH)-K(H ) resonances observed in the 1 H, 1 H-NOESY spectrum. How to cite this article: Fallas, J. A. & Hartgerink, J. D. Computational design of self-assembling register-specific collagen heterotrimers. Nat. Commun. 3:1087 doi: 10.1038/ncomms2084 (2012).